A nanometre-scale resolution interference-based probe of interfacial phenomena between microscopic objects and surfaces Interferometric techniques have proven useful to infer proximity and local surface profiles of microscopic objects near surfaces. But a critical trade-off emerges between accuracy and mathematical complexity when these methods are applied outside the vicinity of closest approach. Here we introduce a significant advancement that enables reflection interference contrast microscopy to provide nearly instantaneous reconstruction of an arbitrary convex object’s contour next to a bounding surface with nanometre resolution, making it possible to interrogate microparticle/surface interaction phenomena at radii of curvature 1,000 times smaller than those accessible by the conventional surface force apparatus. The unique view-from-below perspective of reflection interference contrast microscopy also reveals previously unseen deformations and allows the first direct observation of femtolitre-scale capillary condensation dynamics underneath micron-sized particles. Our implementation of reflection interference contrast microscopy provides a generally applicable nanometre-scale resolution tool that can be potentially exploited to dynamically probe ensembles of objects near surfaces so that statistical/probabilistic behaviour can be realistically captured. Deformation of soft micron-sized particles near surfaces is fundamentally important in fields ranging from colloid science to biomedicine [1] , [2] , [3] , [4] , [5] , [6] , [7] . However, these phenomena are challenging to directly probe, because the corresponding deformation dynamics often cannot be resolved with sufficiently high spatial and temporal resolution. An experimental technique that has shown particular promise involves illuminating an object in close proximity to a surface from below using monochromatic light. Interference of light reflected back from different optical interfaces in the system directly reveals the existence of contact phenomena, if any, while the characteristic fringe pattern that emerges inherently embeds detailed information about the object’s shape near the substrate at up to a microsecond-scale temporal resolution [8] . Reflection interference contrast microscopy (RICM) [9] , [10] , [11] employs non-planar interface image formation theory as a basis to extract this information and accurately reconstruct the surface profile, but its mathematical complexity renders the model cumbersome to implement in its full form [12] , [13] , [14] , [15] , [16] . These difficulties have stimulated development and continuous use of approaches that simplify the connection between the object’s shape and the spacing between neighbouring fringes in the interferogram [10] , [17] , [18] , [19] , [20] , [21] . But this simplicity is achieved at the expense of reconstruction accuracy, particularly when applied to curved microscopic objects, because these methods are strictly valid only for the case of planar parallel interfaces. In this work, we have devised a hybrid approach that couples a simplified non-planar RICM model with an innovative analysis of the entire interferogram; as a result, an arbitrarily shaped convex object can be accurately reconstructed with an unprecedented nanometre-scale resolution. Direct imaging of contact phenomena Our approach provides an extraordinary accurate picture of microparticle–surface interaction phenomena that greatly enhances well-known RICM capabilities extensively applied in the study of particle, cell and lipid/polymer vesicle adhesion [17] , [22] , [23] , [24] , [25] , [26] , [27] , [28] . However, this technique has seen limited application in other fields where the great potential behind RICM’s high resolution, set-up simplicity and unique non-invasive ‘view-from-below’ perspective can produce a significant impact. This becomes evident by comparing the RICM images obtained from polystyrene latex (PSL) particles deposited on a glass substrate under different conditions. Qualitatively, no significant particle deformation and a finite separation distance from the substrate are seen when dry particles are directly deposited on the surface (dry deposition, Fig. 1a ) and observed within a few hours, as indicated by interferograms that display a clean uniform pattern of concentric rings without a minimum intensity value at the centre. But some RICM images significantly change when the particles are deposited evaporatively from solution (wet deposition) and observed after more than 24 h. Here the concentric ring pattern no longer extends to the centre of the interferogram, but terminates at a finite radius outlining what looks like a contact area with a non-homogeneous intensity ( Fig. 1b ). Scanning electron microscopy (SEM) images also reveal significant changes in the contact region due to the water meniscus and accompanying capillary forces imposed during drying [29] , [30] . The extreme nature of these forces is especially evident in visible rugosity, in some cases appearing as if material has been pulled away from the particle surface. The interferograms become further distorted when impurities in the deposition solution accumulate around the perimeter of the contact zone ( Fig. 1c ). Although the interference fringe patterns become difficult to distinguish, the shape and extent of the surrounding deposition region can be quantified. 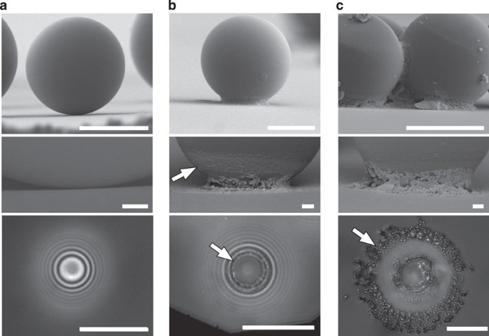Figure 1: RICM reveals different particle deposition scenarios. Dry (a) and wet (b,c) deposition of 15-μm diameter PSL particles on a glass substrate studied with SEM (top/middle; scale bar, 10/1 μm) and RICM (bottom; scale bar, 10 μm). Contrary toa, a contact region with a non-uniform appearance and substantial rugosity in the SEM (arrow) are seen inb, and these non-unformities become magnified when impurities accumulate underneath and around the particles inc. In bothbandc, the RICM images clearly show the shape and extent of these features (arrows). Figure 1: RICM reveals different particle deposition scenarios. Dry ( a ) and wet ( b , c ) deposition of 15-μm diameter PSL particles on a glass substrate studied with SEM (top/middle; scale bar, 10/1 μm) and RICM (bottom; scale bar, 10 μm). Contrary to a , a contact region with a non-uniform appearance and substantial rugosity in the SEM (arrow) are seen in b , and these non-unformities become magnified when impurities accumulate underneath and around the particles in c . In both b and c , the RICM images clearly show the shape and extent of these features (arrows). Full size image RICM also enables direct observation of liquid water underneath larger glass beads ( Fig. 2a ), as evident by a continuously shrinking meniscus due to drying following wet deposition ( Fig. 2b ) and visible motion of the meniscus boundary when an external air flow is imposed ( Supplementary Movie 1 ). Unexpectedly, a distinct meniscus remains evident even after 72 h of drying under vacuum. Hence, RICM directly reveals, for the first time and to the best of our knowledge, the presence of small amounts of water (volumes in the order of 1 fl owing to capillary condensation [30] ) underneath micron-sized particles after dry deposition on a glass substrate and upon exposure to ambient conditions for several days ( Fig. 2c ). 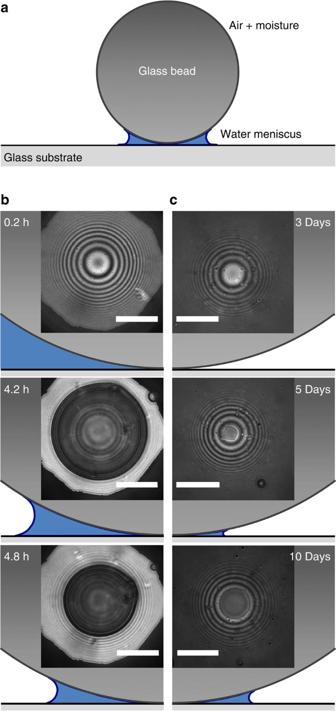Figure 2: RICM observation of a liquid meniscus between micron-sized particles and a substrate. (a) Schematic representation of the water meniscus between 30 to 60 μm diameter glass beads and a glass surface. Following wet deposition, a meniscus forms and shrinks due to evaporation (b), whereas a few days after dry deposition this interfacial water appears and increases by condensation under ambient conditions (20 °C, 51% relative humidity) (c). Menisci illustrations inbandcare not drawn to scale; scale bar, 10 μm in RICM images. Figure 2: RICM observation of a liquid meniscus between micron-sized particles and a substrate. ( a ) Schematic representation of the water meniscus between 30 to 60 μm diameter glass beads and a glass surface. Following wet deposition, a meniscus forms and shrinks due to evaporation ( b ), whereas a few days after dry deposition this interfacial water appears and increases by condensation under ambient conditions (20 °C, 51% relative humidity) ( c ). Menisci illustrations in b and c are not drawn to scale; scale bar, 10 μm in RICM images. Full size image Fringe-spacing analysis based on simplified non-planar RICM Although contact phenomena can be directly observed and quantified (typically as an area in the RICM image), accurate analysis of the interference pattern requires a link between the intensities and the object’s geometry ( Fig. 3 ). Instead of applying the complete non-planar interface image formation theory, where all possible contributions to the observed intensity must be individually determined [16] , we consider a simplified two-dimensional model whereby a single set of complementary rays, I 0 , interfere to produce the intensity observed at a position x in the interferogram, I ( x ). For the single-layer system in Fig. 4a , I ( x ) depends on the interference of rays I 1 and I 2 in terms of their optical path length difference OPLD (term in square brackets) as follows. 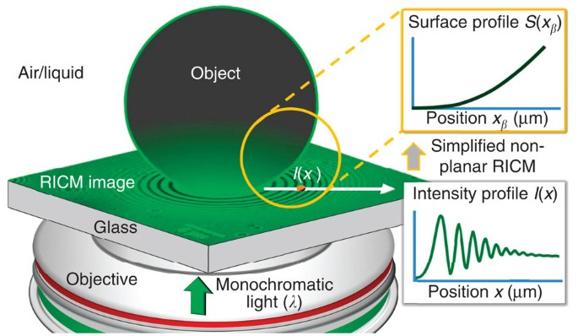Figure 3: Schematic of surface profile reconstruction. Interference fringe patterns obtained from RICM images embed precise information about an object’s topography in the vicinity of contact with a surface. Figure 3: Schematic of surface profile reconstruction. Interference fringe patterns obtained from RICM images embed precise information about an object’s topography in the vicinity of contact with a surface. 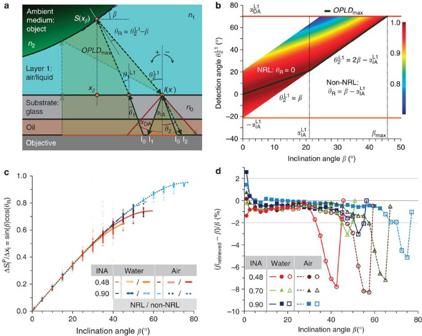Figure 4: Fringe-spacing analysis based on simplified non-planar RICM. (a) Simplified non-planar RICM image formation model. The intensityI(x) is produced by the interference of raysI1andI2, which correspond to the single set of complementary raysI0with the maximumOPLD(determined by geometric parametersS(xβ),βandθRdefined at positionxβ) among all possible contributions (shaded area). ComplementaryI0originate from within the illumination cone (θ1≤αIA, whereαIAis given by the illumination numerical aperture, INA, of the microscope); then, they are reflected back from planar (substrate/layer 1 atx) and non-planar (layer 1/object atxβ) interfaces producing raysI1andI2, respectively, which interfere at positionxonly if they are incident within the cone of detected light (θ2≤αDA, whereαDAis determined by the numerical aperture, NA, of the objective). (b) The formulation of the simplified non-planar RICM model is completed when NRL/non-NRL regimes are identified atOPLDmax, as illustrated with a normalizedOPLDplot for the range of detection angles corresponding to a series of wedge inclination angles with INA=0.48 and water surroundings. (c) Despite the intrinsic fringe-spacing variability, which produces the scattered data points, the behaviour of ΔSPf/Δxfwith inclination angle observed in simulations from several different wedge systems is in excellent agreement with equation (4), where INA,n1(surroundings composition) andθR(reflected light regime) are the main parameters. (d) Percentage error of inclination angles retrieved from the averages of all fringe-spacing values originated from simulations of comparable wedge systems. Closed and open symbols representβretrieved, using NRL and non-NRL models, respectively. In all figures, simulations are performed with numerical aperture=1.25 for wedge angles ranging from 0° toβmax. Full size image Figure 4: Fringe-spacing analysis based on simplified non-planar RICM. ( a ) Simplified non-planar RICM image formation model. The intensity I ( x ) is produced by the interference of rays I 1 and I 2 , which correspond to the single set of complementary rays I 0 with the maximum OPLD (determined by geometric parameters S ( x β ), β and θ R defined at position x β ) among all possible contributions (shaded area). Complementary I 0 originate from within the illumination cone ( θ 1 ≤ α IA , where α IA is given by the illumination numerical aperture, INA, of the microscope); then, they are reflected back from planar (substrate/layer 1 at x ) and non-planar (layer 1/object at x β ) interfaces producing rays I 1 and I 2 , respectively, which interfere at position x only if they are incident within the cone of detected light ( θ 2 ≤ α DA , where α DA is determined by the numerical aperture, NA, of the objective). ( b ) The formulation of the simplified non-planar RICM model is completed when NRL/non-NRL regimes are identified at OPLD max , as illustrated with a normalized OPLD plot for the range of detection angles corresponding to a series of wedge inclination angles with INA=0.48 and water surroundings. ( c ) Despite the intrinsic fringe-spacing variability, which produces the scattered data points, the behaviour of Δ S P f /Δ x f with inclination angle observed in simulations from several different wedge systems is in excellent agreement with equation (4), where INA, n 1 (surroundings composition) and θ R (reflected light regime) are the main parameters. ( d ) Percentage error of inclination angles retrieved from the averages of all fringe-spacing values originated from simulations of comparable wedge systems. Closed and open symbols represent β retrieved , using NRL and non-NRL models, respectively. In all figures, simulations are performed with numerical aperture=1.25 for wedge angles ranging from 0° to β max . Full size image Here β is the inclination angle of the non-planar interface at position x β relative to the horizontal plane, S ( x β ) is the object’s local height above the substrate at x β , θ R is the angle of reflection at S ( x β ), λ =546 nm is the wavelength of the illuminating light (only monochromatic green light is considered here), n 1 is the refractive index of layer 1 (L1) and δ accounts for a phase shift of π if the refractive index of the object is higher than the index of the medium. Therefore, the intensity at x can be determined using geometric parameters S ( x β ), β and θ R at any appropriate x β , where the following relationship, from the geometry in Fig. 4a , is satisfied: The ensemble of admissible x β is bounded by the range of incident angles within the illumination and detection cones ( α IA and α DA , respectively), according to the complete non-planar RICM theory. By identifying the single set of complementary rays making the most significant contribution to I ( x ) within these constraints, our analysis seeks to establish a bijective mapping between x and x β applicable to the whole range of conditions where interference occurs. In contrast, previous simplified models formulated since the early stages of RICM have seen their accurate implementation limited to interfaces with small inclinations and/or small illumination numerical aperture (INA) values, because they neglect non-planar effects ( β =0) and/or assume that only normal incidence light ( θ R = β ) is important [9] , [10] , [21] , [31] , [32] . To envision this, we first consider a wedge geometry ( β =constant) in which case OPLD =2 n 1 sin( β )cos( θ R ) x . The cosine dependence in OPLD implies that the most significant contribution to I ( x ) occurs when OPLD is maximized; hence, our analysis is set at a given β , x and n 1 , leaving cos( θ R ) as the remaining unknown. Although this term displays a maximum at θ R =0, the admissible values are constrained by the finite range of allowable illumination and detection angles ( Fig. 4b ). When β < α IA,L1 , OPLD max occurs when θ R =0 (the normal reflected light (NRL) regime). For α IA,L1 ≤ β ≤ β max =( α IA,L1 + α DA,L1 )/2, however, the set of rays corresponding to θ R =0 no longer contribute to I ( x ). Here the angle θ R associated with OPLD max is a function of β with θ R = β − α IA,L1 (the non-NRL regime). These regimes establish a map from β to θ R and, therefore, a bijective mapping between x and x β at OPLD max (see Supplementary Fig. S1 , Supplementary Table S1 and Supplementary Note 1 ). To make the formulation more suitable for practical implementation, first equation (1) is rewritten in terms of experimentally measurable maximum and minimum intensities, I max and I min , respectively, and a height value S P is expressed as a function of I ( x ) according to conventional inverse cosine transform methods. Here A =( I max + I min )/2, B =( I max − I min )/2, Δ S P f = λ /4 n 1 and δ = π for all cases studied. Notice that S P = S ( x β ) only when planar parallel interfaces and normal incidence light are assumed ( β = θ R =0), and Δ S P f represents the constant height increment between two consecutive fringes. Then, using a wedge geometry (that is, where β and θ R are both position independent), equation (2) and equation (3) are applied to any two intensities with a spacing Δ x and located on a common branch of the intensity profile (that is, between the successive extrema that determine I max and I min ) taken along the direction perpendicular to the fringe’s front in the RICM image, so that the inclination angle β can be related to the corresponding measured increments Δ S P and Δ x (see Supplementary Fig. S2 and Supplementary Methods ). To verify this relationship, we next cast our analysis in terms of Δ x as the spacing between neighbouring fringes in the interferogram Δ x f −a convenient parameter to extract experimentally; in this case, Δ S P =Δ S P f is constant. The complete non-planar interface image formation theory is used to simulate fringe spacings as a function of β in wedge systems under an ensemble of different refractive index and illumination conditions for single- and double-layer objects in both air and water surroundings (see Supplementary Table S2 ). Up to 51 individual fringes are computed for each case to account for intrinsic variability associated with Δ x f in a given wedge system. These data superimpose when coplotted, thereby establishing a mapping from β to Δ S P f /Δ x f that is successfully reproduced by equation (4) when the appropriate reflected light regimes are used ( Fig. 4c ). Then, hundreds of Δ S P f /Δ x f values corresponding to comparable systems (that is, the same β , n 1 and INA) are averaged to perform an inverse mapping (from Δ S P f /Δ x f to β retrieved ) by means of equation (4), to evaluate the accuracy of the fringe-spacing analysis, as the original β is known ( Fig. 4d ). The values of β retrieved are in excellent agreement with those used in the simulations of the complete non-planar theory up to a cut-off value of β * corresponding to the midpoint of the non-NRL regime in Fig. 4b . Therefore, equation (4) enables direct measurement of inclination angles of wedge-shaped interfaces (from 0° to β * ), such as small contact angles of liquid droplets, avoiding the use of fittings or angular correction factors based on full non-planar theory calculations [15] , [16] , [33] . Near-instantaneous surface profile reconstruction We now seek to apply these insights developed for wedges of constant β , toward analysis of intensity profiles corresponding to convex geometries with spatially varying inclination angles. 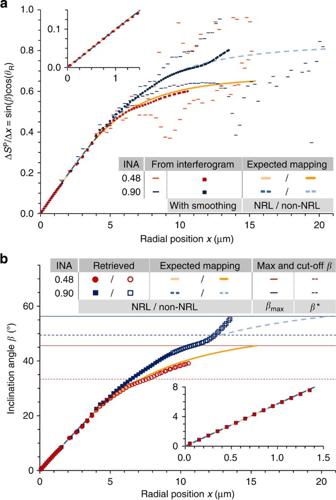Figure 5: Convex geometry analysis. (a) Simulated ΔSP/Δxversusxmapping corresponding to a 10 μm radius sphere in water contacting a glass substrate with numerical aperture=1.25 and glass/water/particle refractive indices of 1.53/1.33/1.55, respectively. (b) Retrieved inclination angles from smoothed ΔSP/Δxare cut off atβ*, because significant errors are obtained beyond this value. Given that the geometry is known, it is possible to determine the expected mappings between the studied variables according to the NRL/non-NRL models. Figure 5a shows Δ S P /Δ x for a spherical particle as a function of radial position from the centre of the fringe pattern x obtained from interferograms simulated using the complete non-planar interface image formation theory. To generate this mapping, two different but complementary transformations of the intensity data are performed: first, for radial positions less than the location of the first intensity extrema, neighbouring intensity values are analysed so that Δ x is constant, and Δ S P is calculated using equation (3) ( Fig. 5a inset), and second, for those positions where interference fringes exist, Δ x is taken as the fringe spacing Δ x f and Δ S P =Δ S P f , exactly as in the previously discussed wedge case (for more details see Supplementary Methods ). As a result, the relationship between Δ S P /Δ x and x from the first transformation follows a clear and smooth trend, although for experimental interferograms some variability is expected because of noise in the intensity values. The data from the second transformation is not as clearly defined as the Δ S P f /Δ x f versus β data for the wedge case ( Fig. 4c ), especially as radial position increases, because a single fringe spacing now incorporates contributions from multiple values of β at different locations on the object’s contour (in addition to the intrinsic variability observed in Δ x f for a particular β ). A general trend can be established, however, by applying a smoothing procedure subject to the constraints that the smoothed Δ S P /Δ x data must increase monotonically with x , and according to equation (4) there is a maximum value that corresponds to β max . Figure 5: Convex geometry analysis. ( a ) Simulated Δ S P /Δ x versus x mapping corresponding to a 10 μm radius sphere in water contacting a glass substrate with numerical aperture=1.25 and glass/water/particle refractive indices of 1.53/1.33/1.55, respectively. ( b ) Retrieved inclination angles from smoothed Δ S P /Δ x are cut off at β *, because significant errors are obtained beyond this value. Given that the geometry is known, it is possible to determine the expected mappings between the studied variables according to the NRL/non-NRL models. Full size image Figure 5a reveals that the smoothed Δ S P /Δ x values closely follow the expected continuous mapping from x to sin( β )cos( θ R ) given by the geometry under consideration and the normal/non-NRL regimes. This indicates that the simplified non-planar RICM model and equation (4) can be successfully applied to interferograms from convex geometries to accurately retrieve the inclination angles β associated with Δ S P and Δ x increments at discrete values of x ( Fig. 5b ). A logical approach to use this information would be to approximate the unknown surface profile of the object as an ensemble of wedges (shown for a spherical object in Supplementary Fig. S1 , where the intensity at each point in the interferogram is successfully mapped to a corresponding value of β ). But it is challenging to use Δ S P , Δ x and the retrieved β -values alone to perform an accurate surface profile reconstruction, because Δ x is inherently large (that is, fringe spacing), limiting the resolution by which the profile can be discretized, a current issue with simplified formulations that directly map fringe spacing to a constant incremental change in the object’s local height above the substrate [9] , [10] , [21] . To overcome these limitations, a continuous approach to the problem is formulated. The discrete mapping between x and β in Fig. 5b is used to define β as a continuous function of x and, therefore, θ R as a function of x . Then, the bijective mapping between x and x β that is necessary to reconstruct the object’s surface profile is achieved by using the geometrical relationship in equation (2) to obtain the following first-order ordinary differential equation (see Supplementary Methods ). The initial condition x β 0 corresponding to the position x 0 of the first Δ S P /Δ x data point is determined from equation (2), where β ( x 0 ) and θ R ( x 0 ) are given by the previously defined mappings, and a slightly modified equation (4) (to account for an additional phase-shift factor S* when multiple layers are present [34] ) provides S ( x β 0 ). The differential equation is straightforward to solve with the minimal computational effort (for example, using MATLAB on an ordinary desktop personal computer) and a continuous surface profile is obtained by reorganizing equation (2) in the form S ( x β ) versus x β . We validated our simplified reconstruction approach using experimentally obtained interferograms from the RICM analysis of a glass bead in air and polymer vesicles in aqueous medium, which are in close proximity to a glass substrate ( Fig. 6 ; INA=0.48 and numerical aperture=1.25). The optical path in the glass bead system is composed of glass/air/glass media with refractive indices of 1.53/1/1.51, respectively. The polymer vesicle systems involve glass/buffer/polymer membrane (15-nm thickness [35] )/sucrose solution with refractive indices of 1.53/1.334/1.51/1.351, respectively. 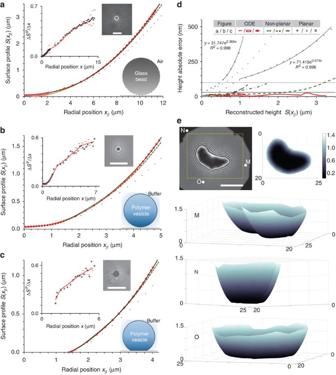Figure 6: Near-instantaneous surface profile reconstruction. Detailed surface profile reconstruction of a glass bead in air (a) and polymer vesicles in buffer solution hovering next to the substrate (b) and in contact with the substrate (c); insets present the corresponding RICM images (scale bar, 10 μm), schematic representations of the system and ΔSP/Δxversusxfrom a simulated non-planar fit (black exes) to experimental data (light red symbols/line, without/with smoothing). Four different procedures (listed in increasing order of accuracy) are used to reconstruct the bottom shape of these specimens: discrete planar (gray dots) and non-planar (dashed green line) methods, continuous ODE (closed/open red circles, NRL/non-NRL) approach and non-planar fit (thin black line). A sphere profile (thick orange line) is fitted to selected reconstructed heights from the ODE method and the non-planar fit is used to define the expected surface profile so that the error of the other procedures can be quantified (d). (e) A three-dimensional reconstruction of the bottom shape of a non-symmetric polymer vesicle hovering next to the substrate (~37 nm) as observed from three different points of view approximately located at M, N and O in the RICM image, with the corresponding bottom view also shown; heights in the colour bar and positions are given in microns, scale bar, 10 μm in the RICM image. Figure 6: Near-instantaneous surface profile reconstruction. Detailed surface profile reconstruction of a glass bead in air ( a ) and polymer vesicles in buffer solution hovering next to the substrate ( b ) and in contact with the substrate ( c ); insets present the corresponding RICM images (scale bar, 10 μm), schematic representations of the system and Δ S P /Δ x versus x from a simulated non-planar fit (black exes) to experimental data (light red symbols/line, without/with smoothing). Four different procedures (listed in increasing order of accuracy) are used to reconstruct the bottom shape of these specimens: discrete planar (gray dots) and non-planar (dashed green line) methods, continuous ODE (closed/open red circles, NRL/non-NRL) approach and non-planar fit (thin black line). A sphere profile (thick orange line) is fitted to selected reconstructed heights from the ODE method and the non-planar fit is used to define the expected surface profile so that the error of the other procedures can be quantified ( d ). ( e ) A three-dimensional reconstruction of the bottom shape of a non-symmetric polymer vesicle hovering next to the substrate (~37 nm) as observed from three different points of view approximately located at M, N and O in the RICM image, with the corresponding bottom view also shown; heights in the colour bar and positions are given in microns, scale bar, 10 μm in the RICM image. Full size image Our method enables reconstructed surface profiles to be obtained near-instantaneously (~1 s of computation time) from the corresponding interferograms ( Fig. 6a–c ). For comparison, two of these contours are obtained by means of discrete non-planar (using arbitrary small increments, see Supplementary Methods ) and planar (traditional analysis [9] , [10] ) methods, and a third one is computed after solving the ODE in equation (5). The accuracy of these near-instantaneous procedures is then verified by comparing their predictions with the most accurate analysis available, using the full non-planar model of RICM [16] requiring ~1 h of computation time (non-planar fit in Fig. 6a–c ). Figure 6d clearly indicates that the continuous approach of the ODE method produces the best results with an error that does not have a tendency to increase as the reconstructed height increases, and, in general, is smaller than 30 nm (black dashed line) over the entire range of intensities analysed (essentially including all available fringes up to the 30th, 22nd and 17th fringes for the results in Fig. 6a–c , respectively). Of the discrete approaches, only the non-planar formulation maintains a similar degree of accuracy for a significant portion of the reconstructed heights, although the error increases to about 100 nm (black dotted line) at the end. For the discrete planar method, the error can grow quickly and even exponentially (the contour is underpredicted), especially when errors are larger than 100 nm. This description of the error closely resembles the behaviour observed in simulated systems (see Supplementary Fig. S3 and Supplementary Note 2 ). Fundamental quantitative descriptors of an object’s deformation can be easily obtained from the reconstructed profiles. As symmetry in the RICM images and bright-field observation suggest that the systems in Fig. 6a–c adopt an overall spherical shape, fitting the predicted contours based on a spherical geometry yields estimated radii, R sphere , and height values at the centre of the symmetric interferograms, S sphere 0 (see Supplementary Fig. S4 , Supplementary Table S3 and Supplementary Discussion ). R sphere of 21.13, 8.51 and 7.12 μm for the glass bead, suspended vesicle and vesicle in contact with the substrate, respectively, are in close agreement with corresponding values of 21.55, 8.38 and 7.23 μm, measured directly from the bright-field images, confirming an overall spherical shape (truncated sphere for the vesicle in contact, as assumed theoretically [36] , [37] and shown with confocal microscopy [38] ). S sphere 0 values determined from the fitting provide from qualitative to quantitative information on each particular case. For the glass bead, RICM shows a finite separation distance of 49±1 nm between particle and substrate, likely attributable to surface roughness [39] , [40] , [41] , [42] , which compared with a negative S sphere 0 of −22.6 nm points to significant deviations from a perfectly spherical geometry at the nanoscale. An approximately spherical shape is maintained by the vesicle hovering near the substrate with deformation only observed within 250 nm above the glass, as indicated by the spherical fitting and a positive S sphere 0 of 32.2 nm close to that measured directly from RICM (41±1 nm). For the vesicle in contact, a negative S sphere 0 of −138.2 nm allows the calculation of a 1.396-μm contact radius and a 11.3° contact angle based on a truncated sphere geometry, in excellent agreement with the corresponding measurements from RICM (1.4 μm and 9.9° at a height of 7 nm). A contact radius to vesicle radius ratio of ~0.2 is close to previous reported values for similar shell-polymerized vesicles in contact with a glass substrate [38] . Material deformation of soft micron-sized objects at surfaces is fundamentally important in a host of fields, but these effects have proven challenging to probe experimentally. It has long been appreciated that RICM enables the vicinity of a contact region between a microscopic object and a bounding surface to be characterized with nanometric resolution, but a complete accurate implementation of the technique to study dynamic phenomena has been challenging. The analysis of RICM interferograms introduced here overcomes many of these limitations, simultaneously incorporating all fringes available from the set-up resolution in a fast and accurate reconstruction of the non-contact regime surface profiles. Our results validate the method under diverse experimental conditions (air/aqueous media) and different characteristics of the reflecting surface (smooth, soft polymer vesicle membrane versus rougher, solid glass bead), and Fig. 6e clearly indicates that it is applicable to arbitrarily shaped convex objects. In addition, RICM experiments reveal topologically complex local deformations and contact phenomena relevant to virtually all adhesion models. The finding of various scenarios at the micro scale after dry/wet deposition of PSL particles on a glass substrate is in qualitative agreement with recent results that show how different deposition media affect the particle removal efficiency, a fact attributed to plastic deformation of particles caused by capillary forces [43] . Even more significant is the direct observation of femtolitre-scale capillary condensation dynamics underneath micron-sized particles, believed to be unique, given that capillary condensation have only been directly observed using environmental SEM [44] , [45] and studied with the surface forces apparatus [46] , [47] , although employing two crossed cylindrical mica surfaces with very large radii of curvature (~1–2 cm). This unparalleled view of the particle–substrate interface offered by RICM reveals new details corresponding to more realistic conditions (different particle deposition scenarios, humidity effects and accurate contour reconstruction), while potentially enabling near real-time analysis of ensembles containing hundreds of particles near surfaces so that statistical/probabilistic behaviour can be realistically captured. Image acquisition The microscope set-up employed in our experiments was a Zeiss Axiovert 200M inverted microscope. Monochromatic green light, 546.1 nm, was obtained from a 103W HBO mercury vapour lamp using a 5-nm band-pass filter. The microscope was equipped with a Zeiss Antiflex EC Plan-Neofluar × 63/1.25 Oil Ph3 objective and RICM images were recorded with a Zeiss AxioCam MRm camera. SEM images were taken by Dr Yordanos Bisrat at the Materials Characterization Facility at Texas A&M University, using an ultra-high-resolution field-emission SEM, the JEOL JSM-7500F. Sample selection and preparation The experimental systems chosen for testing our surface profile reconstruction procedure are a glass bead and three cross-linked polymer vesicles [48] close to a glass substrate. There are several reasons for this sample choice. First, bright-field observation and the symmetry in the RICM images indicate that the glass bead and two of the polymer vesicles clearly adopt an overall spherical shape (see Supplementary Fig. S4 ), whereas the third polymer vesicle presents a non-symmetric RICM image ( Fig. 6e ) that corresponds to an arbitrary convex geometry. The second one is the objects’ geometry at their bottom. Polymer vesicles (which are perfectly spherical when free in solution) are expected to experience deformation when close to or in contact with a planar surface. The glass bead, although hard to deform despite being in contact with the substrate, might offer other interesting effects such as surface roughness and a close look to its assumed spherical shape. The third aspect is the objects’ surfaces, where the vesicles represent added complexity because of the presence of the smooth polymer membrane (double-layer system), when compared with the rougher glass bead surface (single-layer system). Finally, the polymer vesicles are in aqueous surroundings while the particle is in air, verifying the applicability of the procedure under different experimental conditions. Block copolymer vesicles spontaneously form in water when the copolymer has one hydrophobic and one hydrophilic block, called amphiphilic diblock copolymers [49] , [50] . We used polyethylene oxide-block-polybutadiene (PEO 89 PBd 120 , molecular mass 10,400 g mol −1 ) purchased from Polymer Source Inc. (Canada). For vesicle preparation, a polymer film containing 250 μg of the block copolymer is formed by evaporation (8 h) at the bottom of a 5-ml glass scintillation vial and the film is rehydrated during 24 h at 60 °C with 1–2 ml of a 300 mOsm kg –1 sucrose solution (Osmometer model 3320, Advanced Instruments, Inc., Norwood, MA). To obtain shell-polymerized vesicles, the resulting solutions were exposed for 1–3 h to 200 μl of 20% ammonium persulphate (99%) and 30 μl of 1,2-bis(dimethylamino)ethane (99%). Then, the vesicles are placed in phosphate buffered saline (PBS) solution of equal osmotic pressure than their interior. Ammonium persulphate and 1,2-bis(dimethylamino)ethane were obtained from Acros Organics (Morris Plains, NJ), whereas PBS and sucrose (ACS reagent) were purchased from Fisher Scientific (Pittsburgh, PA). On the other hand, the glass beads used are obtained from Polysciences Inc. (USA); they come in powder form and are made of soda lime glass. In the dry/wet deposition experiments reported in Fig. 1 , SEM images correspond to 15-μm diameter fluorescent green PSL particles purchased from Thermo Fisher Scientific Inc. (USA) in powder form. A 5-nm coating of platinum/palladium was applied when necessary for SEM observation. PSL particles are used, because their smooth surface is expected to reveal the effects of strong capillary forces acting during drying. RICM experiments and image analysis A droplet of vesicle solution and dry/wet particles are placed directly on top of an optical borosilicate cover glass (0.16–0.19 mm thickness) for bright-field and RICM observation. To obtain polymer vesicles hovering next to the substrate, the cover glass is previously treated with bovine serum albumin (BSA) to avoid adhesion and spreading of the vesicles onto the glass surface. Processing of RICM images was performed with the software ImageJ 1.41o (public domain, National Institutes of Health, USA) and MATLAB R2010a, and the procedure implemented to extract quantitative information is described in the following. First, a background homogenization routine is executed so that minimum separation distance measurements can be performed accurately. Then, the intensity profile along an observation line is measured or, if there is circular symmetry in the RICM image, the centre of the interferogram is located and a circular average of intensities is obtained, followed by a ‘zero’ intensity subtraction (from the dark area outside the field of view) and normalization by the exposure time. The positions of peaks and valleys (and consequently the fringe spacing) are determined from the resulting intensity profile, so that the surface profile reconstruction procedures can be performed. To obtain an absolute contour reconstruction, the experimental intensity values are scaled to match the simulated intensity versus height curve from the theory for stratified planar structures, and the minimum separation distance between the specimens and the glass is measured assuming that particles and vesicles are close enough to the glass substrate (minimum separation distance <200 nm). How to cite this article: Contreras-Naranjo, J. C. & Ugaz, V. M. A nanometre-scale resolution interference-based probe of interfacial phenomena between microscopic objects and surfaces. Nat. Commun. 4:1919 doi: 10.1038/ncomms2865 (2013).